The draft genome of the large yellow croaker reveals well-developed innate immunity The large yellow croaker, Larimichthys crocea , is one of the most economically important marine fish species endemic to China. Its wild stocks have severely suffered from overfishing, and the aquacultured species are vulnerable to various marine pathogens. Here we report the creation of a draft genome of a wild large yellow croaker using a whole-genome sequencing strategy. We estimate the genome size to be 728 Mb with 19,362 protein-coding genes. Phylogenetic analysis shows that the stickleback is most closely related to the large yellow croaker. Rapidly evolving genes under positive selection are significantly enriched in pathways related to innate immunity. We also confirm the existence of several genes and identify the expansion of gene families that are important for innate immunity. Our results may reflect a well-developed innate immune system in the large yellow croaker, which could aid in the development of wild resource preservation and mariculture strategies. The large yellow croaker (referred to as ‘croaker’ hereafter), Larimichthys crocea , is an economically important marine fish species in China that is largely endemic to coastal waters of the eastern and southern parts of the country [1] . Unfortunately, wild stocks have severely suffered from overfishing in the last few decades [1] . Although artificial mariculture in China has made advances in croaker rearing since 1985, aquacultured croakers are likely to have reduced genetic diversity and disease resistance [2] . Moreover, aquacultured croakers are extremely vulnerable to various marine pathogens, including bacteria (that is, vibrio [3] , nocardia [4] and pseudomonas [5] ), viruses (that is, iridovirus [6] ) and parasites (that is, Cryptocaryon irritans [7] and benedenia [8] ). Outbreaks of infectious diseases and decreased disease resistance in maricultured croaker species have markedly affected the fishery industry [2] . We suspected that the disease vulnerability of croaker might also be due to special genomic and evolutionary patterns of its immune system. Several immune-relevant genes have been studied in a range of teleost species, including croaker [9] . Extensive knowledge has been accumulated that shows the complexity of the teleost innate immune system, whereas information relating to adaptive immunity remains insufficient [10] . Gene expression profile studies of immune processes in croaker [11] , [12] found that genes encoding innate defense molecules such as toll-like receptors (TLRs), interleukins (ILs) and tumour necrosis factors (TNFs) were significantly upregulated after infection. Whole-genome sequencing has uncovered a unique immune system in Atlantic cod ( Gadus morhua ) [13] that lacks genes for MHC class II, CD4 and invariant chain (Ii). However, MHC class I genes are expanded to compensate for the loss of CD4 + T-helper cells [13] . In this study, we examine the entire croaker genome, using next-generation sequencing (NGS) technology to reveal the genome structure and the genes underlying the immune system. Our results could further improve wild croaker protection and mariculture. Genome sequence and assembly We sequenced the genome of a wild-caught female croaker using whole-genome shotgun sequencing. Following the standard protocol (Illumina, San Diego, CA, USA), we constructed sequencing libraries for paired-ends (PE) and mate-pairs (MP) and sequenced them on an Illumina Genome Analyzer II sequencer (GAII). 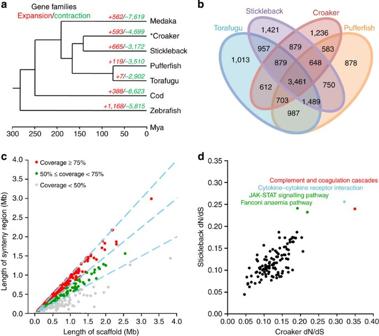Figure 1: Comparison of evolutionary features of croaker and other teleosts. (a) Phylogenetic tree and numbers of gene families under expansion (red)/contraction (green). Mya, million years ago. (b) Venn diagram showing unique and overlapping gene families in croaker, stickleback, torafugu and pufferfish. (c) Length of syntenic regions on each scaffold based on stickleback. Scaffolds are indicated by coverage ≥75% (red solid dots), 50%≤ coverage≪75% (green solid dots) and coverage≪50% (grey solid dots). Three blue dashed lines indicate coverage of 50, 75 and 100%, respectively, from bottom to top. (d) KEGG pathways to which rapidly evolving genes were mapped are indicated by pairs of median dN/dS ratios (black solid dots) in croaker and stickleback; significantly enriched (FDR≪0.05) rapidly evolving genes in KEGG pathways are highlighted for croaker (red solid dots), stickleback (green solid dots) or both (blue solid dots). After data filtering, we obtained 757 million reads with an average length of 74 bp for contig assembly and 516 million 2 × 36 bp pairs for scaffold linking( Supplementary Table 1 ). We estimated the genome size to be 728 Mb according to the frequency distribution of 25-mer ( Supplementary Fig. 1 ), which is similar to a previous estimation of 743 Mb translated from 0.76 pg of DNA content ( C -values) [14] , [15] . Using a de novo assembly strategy, we obtained a total of 51,588 contigs with an N50 of 25.7 kb and 10,271 scaffolds with an N50 of 498.7 kb, of which the longest contig and scaffold were 483 kb and 3.8 Mb, respectively ( Table 1 ). These reads yielded a draft genome with a total length of 644 Mb that covered 88% of the estimated genome size ( Table 1 ). After remapping the PE reads to the final assembly, we obtained more than a 15-fold effective depth across 97.5% of the draft genome. 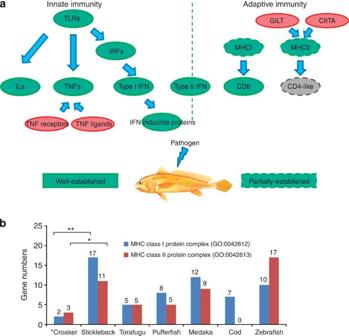Figure 2: Immune characterization of croaker. (a) Proteins encoded by immune-relevant genes in croaker that are present in similar (green circles), higher (red circles) or lower (green circles with dashed outlines) numbers compared with other teleosts, and genes that are absent (grey circles with dashed outlines) in croaker. CIITA=major histocompatibility complex class II transactivator; GILT=gamma-interferon-inducible lysosomal thiol reductase; IFN=interferon; IL=interleukin; IRF=interferon regulatory factor; MHC=major histocompatibility complex; TNF=tumour necrosis factor; TLR=toll-like receptor. (b) Number of genes involved in the cellular component of the MHC class I protein complex (GO:0042612, blue bar) and the MHC class II protein complex (GO:0042613, red bar) in different teleosts. The exact numbers are shown on the top of each bar. The gene numbers in croaker that are significantly lower than those in stickleback are indicated by a single asterisk (P-value=0.08 for GO:0042613) or a double asterisk (P-value=0.0022 for GO:0042612) according to a proportion test. The mean depth of the whole genome is 83-fold ( Supplementary Table 2 ). The assembly metrics of the croaker genome are comparable to those of other teleost genomes, which were generated using an NGS technology [13] , [16] . Table 1 Genome assembly metrics of croaker. Full size table Genome content and annotation We annotated the repeat sequences against the teleost libraries. Analysis revealed that 16.38% of the croaker genome is composed of repeat sequences ( Supplementary Table 3 ), which is ~17.5% in medaka ( Oryzias latipes ) [17] , 11.2% in torafugu ( Takifugu rubripes ) [18] , 25.2% in stickleback ( Gasterosteus aculeatus ) [16] , 25.4% in Atlantic cod [13] and 27.71% in coelacanth ( Latimeria chalumnae ) [19] . Among the classified repeat elements, DNA elements are most abundant in the croaker genome (2.96%), which is similar to that in medaka (3.1%) [17] ; simple repeats occupy 2.39% of the genome, showing the second largest proportion of known repeat sequences, which is much greater than the percentage in torafugu (1.86%) [18] , coelacanth (1.09%) [19] and medaka (0.6%) [17] . In addition, unclassified repeat sequences comprise 7.44% of the croaker genome, almost reaching the proportion of total known repeat sequences (8.94%), which is lower than the proportions in medaka (9.2%) [17] and coelacanth (13.6%) [19] . In general, the proportions of croaker repeat sequences are comparable to those of other teleost fishes. We annotated protein-coding genes as well as non-coding regions using the repeat masked genome ( Supplementary Table 4 ). We predicted 19,362 protein-coding genes containing 186,960 exons in 35 Mb of the draft genome, with an average of 9 exons and 1,491 bp of coding DNA sequencing (CDS) per gene, which is comparable to the metrics of other teleost fishes ( Supplementary Table 5 ). Among the identified protein-coding genes, 16,460 genes had at least one InterPro (IPR) entry [20] ; 13,095 genes were annotated to at least one Gene Ontology (GO) term [21] and 4,671 genes were mapped to 331 Kyoto Encyclopedia of Genes and Genomes (KEGG) pathways [22] ( Supplementary Fig. 2 ). We identified 2.46 million heterozygous single-nucleotide polymorphisms (SNPs) in croaker and validated 75 heterozygous SNPs in 80 randomly selected SNPs ( Supplementary Fig. 3 and Supplementary Table 6 ). With a false discovery rate (FDR) of 6.25%, the estimated rate of heterozygosity was 3.58 × 10 −3 across the whole-croaker genome (644 Mb), which is relatively higher than that of coelacanth (2.80 × 10 −3 ) (ref. 19 ), Atlantic cod (2.09 × 10 −3 ) (ref. 13 ) and stickleback (1.43 × 10 −3 ) (ref. 16 ), while medaka has the highest SNP rate (0.034) among vertebrate species [17] . It is likely that heterozygote rates in teleost fishes are generally higher than those in humans (0.69 × 10 −3 ) (ref. 23 ). Genome evolution To determine the extent of genetic conservation among teleost fishes, we compared seven teleost fish genomes including croaker, stickleback, Atlantic cod, medaka, torafugu, pufferfish ( Tetraodon nigroviridis ) and zebrafish ( Danio rerio ). We identified 17,362 orthologous gene families shared between at least two teleost species, 1,524 of which were single-copy orthologues shared by all the studied species. Using these single-copy orthologues, we explored the phylogenetic relationships of the seven teleost fishes ( Fig. 1a ). The phylogenetic tree revealed that stickleback (order Gasterosteiformes ) was most closely related to croaker (order Perciformes ) with an estimated divergence time of 142 Myr ago. The order Tetraodontiformes , which torafugu and pufferfish belong to, is only slightly less closely related to croaker ( Fig. 1a ), and the separation was estimated to be 191 Myr ago. We studied the orthologue profiles of the four closely related teleosts (croaker, stickleback, torafugu and pufferfish) ( Fig. 1b ). A total of 3,461 gene families were shared among the four fishes, and stickleback, a close relative, had 5,867 overlapping gene families with croaker. We further explored the syntenic relationship between croaker and stickleback ( Fig. 1c ). From 21,012 pairwise blastp comparisons, we obtained 562 syntenic blocks in the croaker genome, which contained 6,597 orthologous croaker genes. These syntenic blocks spanned 485 scaffolds with a total length of 331 Mb (51.4% of the draft genome). Most syntenic regions have high coverage of the respective scaffolds (407 scaffolds with >50% coverage and 289 scaffolds with >75% coverage), confirming a conservation of synteny between croaker and stickleback ( Fig. 1c ). Figure 1: Comparison of evolutionary features of croaker and other teleosts. ( a ) Phylogenetic tree and numbers of gene families under expansion (red)/contraction (green). Mya, million years ago. ( b ) Venn diagram showing unique and overlapping gene families in croaker, stickleback, torafugu and pufferfish. ( c ) Length of syntenic regions on each scaffold based on stickleback. Scaffolds are indicated by coverage ≥75% (red solid dots), 50%≤ coverage ≪ 75% (green solid dots) and coverage ≪ 50% (grey solid dots). Three blue dashed lines indicate coverage of 50, 75 and 100%, respectively, from bottom to top. ( d ) KEGG pathways to which rapidly evolving genes were mapped are indicated by pairs of median dN/dS ratios (black solid dots) in croaker and stickleback; significantly enriched (FDR ≪ 0.05) rapidly evolving genes in KEGG pathways are highlighted for croaker (red solid dots), stickleback (green solid dots) or both (blue solid dots). Full size image When comparing the six other teleosts, we found 79 croaker-specific gene families containing 171 genes; 44 of the genes could be annotated in 15 known IPR domains ( Supplementary Table 7 ), including three immunoglobulin-related domains (IPR013783: immunoglobulin-like fold, IPR007110: immunoglobulin-like domain and IPR003599: immunoglobulin subtype) of seven, six and six genes, respectively. Although genome annotation identified great numbers of croaker genes involved in these IPR domains (630, 396 and 340, respectively), these unique genes might contribute to a special pattern for immunoglobulin in croaker humoral immunity. Moreover, we uncovered 593 croaker gene families with 1,291 genes after expansion. The most expanded gene family was a zinc-finger protein family, which contains seven genes. One of the genes is similar to the human gene ZNF268 , which is associated with human T-cell leukemia virus type 1, and might influence the T-cell development [24] . We also identified the expansion of several immune-relevant gene families in croaker, which includes the TNF ligand superfamily (three genes), the TNF receptor superfamily (three genes), the gamma-interferon-inducible lysosomal thiol reductase (GILT) family (two genes) and the major histocompatibility complex class II transactivator (CIITA) family (two genes). To study adaptive divergence at the molecular level, we estimated the nonsynonymous-to-synonymous substitution (dN/dS) ratios for croaker and stickleback, with pufferfish as the outgroup, using 3,444 single-copy orthologues from the pairwise comparison of all protein-coding genes shared among these three fishes. Rapidly evolving genes were defined as genes with higher dN/dS ratios than the lineage-specific average dN/dS ratios [25] . We identified 467 and 642 rapidly evolving genes in croaker and stickleback, respectively ( Fig. 1d ). These genes are significantly enriched in complement and coagulation cascades (FDR=2.40 × 10 −4 ) and cytokine–cytokine receptor interaction (FDR=0.0016) pathways involved in the regulation of innate immune response [26] and the interaction of signalling molecules, respectively ( Supplementary Table 8 ). We further found 318 genes under positive selection in croaker and 6 genes that are also significantly enriched in complement and coagulation cascade pathways (FDR=0.037, Supplementary Table 8 ), indicating the accelerated evolution of the innate immune system in croaker. Characterization of the croaker immune system Our results revealed a well-established innate immune system and a partially established adaptive immune system in croaker ( Fig. 2a ). We confirmed the presence of innate immunity-relevant genes encoding TLRs, ILs and TNFs in the croaker genome ( Supplementary Table 9 ), which is consistent with previous studies [11] , [27] , [28] , [29] , [30] . Meanwhile, TNF superfamilies of ligands and receptors showed expansion in croaker, suggesting that innate immunity is strengthened by extra copies of TNF-related genes. Figure 2: Immune characterization of croaker. ( a ) Proteins encoded by immune-relevant genes in croaker that are present in similar (green circles), higher (red circles) or lower (green circles with dashed outlines) numbers compared with other teleosts, and genes that are absent (grey circles with dashed outlines) in croaker. CIITA=major histocompatibility complex class II transactivator; GILT=gamma-interferon-inducible lysosomal thiol reductase; IFN=interferon; IL=interleukin; IRF=interferon regulatory factor; MHC=major histocompatibility complex; TNF=tumour necrosis factor; TLR=toll-like receptor. ( b ) Number of genes involved in the cellular component of the MHC class I protein complex (GO:0042612, blue bar) and the MHC class II protein complex (GO:0042613, red bar) in different teleosts. The exact numbers are shown on the top of each bar. The gene numbers in croaker that are significantly lower than those in stickleback are indicated by a single asterisk ( P -value=0.08 for GO:0042613) or a double asterisk ( P -value=0.0022 for GO:0042612) according to a proportion test. Full size image We also confirmed the existence of MHC class I and MHC class II genes, which have been previously cloned from croaker [31] , [32] as well as other teleosts [33] , [34] , [35] , [36] . Despite the broad existence of genes encoding MHC class molecules, comparative functional annotations showed that the numbers of genes involved in the cellular component of MHC class I protein complex (GO: 0042612) and MHC class II protein complex (GO: 0042613) in croaker are much lower than those in other whole-genome sequenced teleosts ( Fig. 2b , Supplementary Table 10 ). Compared with stickleback, which is most closely related to croaker, the discrepancy of gene numbers is significant ( P -value=0.0022 for GO:0042612 and P -value=0.08 for GO:0042613, proportion test). Notably, previous studies have not reported clones for genes encoding either MHC class I-interacting protein CD8 or MHC class II-interacting protein CD4 in croaker. In our study, we detected genes encoding CD8α and CD8β proteins ( Supplementary Table 9 ), but the gene for CD4 is absent in the croaker genome. Interestingly, we found a fragment predicted to be a truncated CD4-like region in the croaker genome. This predicted CD4-transcript with two CDS regions was validated by Sanger sequencing at the cDNA level and was predicted to have 215 amino acids and to be located in a conserved syntenic block within scaffold 181 ( Supplementary Fig. 4 , Supplementary Table 11 ). Compared with the CD4 gene in different teleost fishes, this CD4-like transcript could only be partially aligned with the complete CD4 mRNA regions ( Supplementary Fig. 4 , Supplementary Table 11 ) and thus seemed to have impaired CD4 function. We then carried out quantitative real-time PCR (qPCR) to detect the expression level of this CD4-like transcript in virus-infected croakers ( Supplementary Table 12 ). As the CD4 molecule is essential for T-cell activation in adaptive immunity, it should be highly upregulated after infection. However, the CD4-like transcript was not significantly differentially expressed in virus-infected croakers ( Supplementary Fig. 5 ), which indicated that the CD4-like gene might not act against viral infection. Therefore, the lack of CD4 function and the lower number of genes encoding MHC class molecules demonstrated that adaptive immunity might not be effective in croaker for fighting specific infections. We propose that the well-established innate immunity as well as the expansion of TNF superfamilies could compensate for the imperfect functionality of adaptive immunity in croaker. Moreover, we observed the expansion of the GILT and CIITA gene families in croaker. Both gene families play an important role in adaptive immunity: GILT reduces thiol bonds in exogenous antigens and exposes buried epitopes for MHC class II (refs 37 , 38 ), and CIITA is a transcriptional regulator for MHC class II (refs 31 , 39 ). Therefore, we presumed that the expansion of these gene families indicated an evolutionary trend for adaptive immunity in croaker. In addition, we found one gene encoding type I interferon (IFN) in the croaker genome, as well as other genes encoding IFN regulatory factors (IRFs) and IFN-inducible proteins ( Supplementary Table 9 ), which were characterized in previous clone studies [38] , [40] , [41] , [42] . Studies of expression profiles in infected croaker also reported highly differential expression of IRF genes [11] , [12] . In mammals, type I IFNs serve as innate antiviral cytokines [43] , and related factors such as IRFs and IFN-inducible proteins are involved in the signal pathway of IFN [44] and play a key role in mediating the innate immune response. In addition, the gene encoding for type II IFN (IFNγ), IFNG , was identified in our study, which is crucial to fighting viral invaders in both innate and adaptive immunity and to potentiating the effects of type I IFNs [43] . In this regard, these findings further support the proposal that, in croaker, innate immunity is integrated and effective and compensates for adaptive immunity. The whole-genome sequencing of croaker provided a comprehensive understanding of the species at the genomic and evolutionary levels and revealed a different immune pattern in croaker. Several important innate immunity genes encoding TLRs, ILs and TNFs are present, and TNF-related gene families have expanded in croaker. Meanwhile, rapidly evolved and positively selected genes are significantly enriched in the complement and coagulation cascades pathway. Adaptive immunity genes encoding CD8α and CD8β proteins are present, and the GILT and CIITA gene families also showed expansion. However, the gene for CD4 might not be intact, and the number of genes for cellular components of MHC class I and II are small compared with other teleosts. It is likely that croaker developed an efficient innate immune system for general antigen resistance, while the partially established adaptive immune system is not very effective at responding to specific antigens. This could be a possible explanation for the vulnerability of croaker to broad marine pathogens. Further investigations should concentrate on identifying other immune-relevant genes, validating gene functions in immune pathways and detecting genetic polymorphisms of immune loci between wild and maricultured croaker populations. Meanwhile, with a large wealth of sequence information available, more features of croaker that could influence survival and production will be discovered, thereby benefiting wild resource recovery and the mariculture fishery industry. Croaker sample and sequencing The sequenced female croaker (weight, ~1 kg; body length, ~40 cm; estimated age, 21 months according to otolith rings) was wild-caught by long-range fishermen in the East China Sea area of Zhejiang Province, representing the Daiqu population [1] . Whole-genomic DNA was extracted from the abdominal muscle using a standard three-step phenol-chloroform extraction. We constructed short insert-size (~200 and 500 bp) paired-end libraries and long insert-size (~2, 5 and 9 kb) libraries ( Supplementary Note 1 ). The libraries were hybridized to the surface of flow cells in a cluster station and subjected to 2 × 76 bp read-length of PE runs on a GAII sequencer (Illumina) based on the manufacturer’s instructions. Genome assembly The raw data were filtered using strict criteria ( Supplementary Note 2 ), and we used cleaned reads to estimate the genome size according to the formula D=M/((L–K+1)/L). Sequencing depth (D) was determined by the peak k-mer depth (M), the k-mer length (K) and the average read length (L) [45] . The 25-mer counts were chosen using Jellyfish [46] , and the estimated croaker genome size is 728 Mb. The cleaned reads with PE libraries were assembled de novo to contigs using ABySS [47] . The k-mer was set at 51 bp, other parameters were set as the default, and contigs shorter than 200 bp were discarded. Reads for MT libraries were chopped to 2 × 36 bp as linkers for scaffolding by SSPACE [48] . The default parameters were set to add the linker information step-by-step from the shortest insert size to the longest. After adding PE libraries into the scaffolds, we assessed the pair insert size and orientation of all the MP libraries and kept only the long insert size of reverse-forward pairs in the MP libraries for subsequent scaffolding. Gapcloser [49] was used to close the gaps in the scaffolds, which eliminated 279,464 gaps covering 69,719,924 bp of a total of 320,781 gaps covering 99,204,443 bp (87%). Gene content and prediction Repeats were annotated using RepeatModeler ( http://www.repeatmasker.org ) and RepeatMasker ( http://www.repeatmasker.org ), combined with the repeat database, RepBase [50] . RepeatModeler was used to predict the novel repeat families, and these families were combined with RepBase to produce the final library, from which RepeatMasker was used to call the consensus repeat sequences. For subsequent gene annotations, the genome was masked from these repeat regions, except for simple repeats. tRNA was scanned across the genome using tRNAscan-SE [51] . microRNA was first blasted against miRBase [52] , and then, the secondary structure was predicted by RNAfold [53] . For each record in the database, only 50 hits with the highest E-values were kept for the second step. ncRNA was first blasted against the Rfam [54] database with an E-value cutoff at 0.01. This database was used to retain only one gene, and Infenal [55] was used to predict the ncRNA gene. The final results were combined in the Ensemble pipeline [56] . We annotated the repeat masked genome to predict protein-coding genes using two pipelines (Ensemble [56] and Maker [57] ) with combined annotation methods of ab initio gene annotation, homology-based gene prediction and transcriptome information ( Supplementary Note 3 ). The Ensemble pipeline was used to predict a gene set purely based on DNA sequences and homology to Uniprot protein sequences. The transcriptome data were used to generate expressed sequence tags (ESTs), which were used in the Maker pipeline. Combined with initial annotation from Ensemble and transcript evidence, an improved protein-coding gene set was generated from Maker. We performed functional annotation for protein-coding genes in the croaker genome. We found homologues for protein-coding genes using blastp (E-value=1 × 10 −5 ) with the SwissProt and Trembl subsets of the Uniprot database [58] . To retrieve biological pathways related to the croaker genome, we obtained KEGG orthologous gene information using the KEGG Automatic Annotation Server (KAAS) [22] with a eukaryote representative set as reference and default parameters, and we linked croaker genes to KEGG pathways using an in-house Perl script. For protein family classification and Gene Ontology analysis, we used InterProScan5 (ref. 20) [20] to query multiple protein sequence and protein domain databases (ProDom, HAMAP, PANTHER, TIGRFAMs, PRINTS, PIRSF, Gene3D, COILS, PROSITE, Pfam, SMART) and retrieved GoSlim information from the InterPro database (v46.0). To investigate specific gene features of croaker, we performed functional annotation with six other sequenced teleost genomes ( Danio rerio (zebrafish), Gadus morhua (Atlantic cod), Gasterosteus aculeatus (stickleback), Oryzias latipes (medaka), Takifugu rubripes (torafugu) and Tetraodon nigroviridis (pufferfish)) using the same procedure mentioned above. Heterozygous SNP detection We remapped usable PE reads to draft genome with the BWA program [59] and used GATK [60] to call SNPs. We filtered SNPs using the following criteria: read depth (DP) >10, quality by depth (QD) >10.0, mapping quality (MQ) >50.0, phred score of strand bias (FS) ≪ 13.0, HaplotypeScore ≪ 13.0, MQRankSum >−1.96 and ReadPosRankSum >−1.96. The rate of heterozygosity was estimated as the density of heterozygous SNPs for the whole genome. Gene families We used TreeFam [61] (v4.0) to define orthologous gene families among croaker and the six other teleosts mentioned above. (1) The longest protein sequence of each gene for the six sequenced teleosts was chosen for each gene. (2) After combination with croaker protein sequences, the proteins were blasted against themselves. Solar was used to conjoin the fragmental alignments for each gene-pair. (3) Hcluster_sg (hierarchical clustering) was used to define the clusters. The minimum edge weight and minimum edge density were set to 5 and 1/3, respectively. (4) We multi-aligned each protein cluster using Muscle [62] and converted the clusters into codon alignments using an in-house Perl script. Orthologous groups were built and inferred using TreeBeST. Data from fourfold-degenerate sites were extracted from the single-copy gene families. Modeltest [63] was used to select the best nucleotide substitution model (GTR+gamma+I). MrBayes [64] was used to reconstruct the phylogenetic tree from 1,524 single-copy gene families, which were present in all seven teleost species. The MCMCtree program implemented in PAML [65] was used to predict the divergence time for yellow croaker and other teleosts. Calibration time was obtained from the TimeTree database ( http://www.timetree.org/ ). We used the divergence time of torafugu and pufferfish as the external calibration time (69.8 Myr ago). CAFÉ [66] (v2.0) was used to identify gene families under expansion or contraction. The syntenic relationship between croaker and stickleback was identified using MCScan [67] (v0.8). The lengths of alignment regions were calculated for all scaffolds. Evolutionary analyses To identify rapidly evolving genes, 3,587 single-copy gene families shared within croaker, stickleback and pufferfish were used, and after filtering dS saturation (dS ≥2), 3,444 orthologues remained for analysis. The lineage-specific dN/dS ratios were estimated by concatenating 200 random genes, which were used as the average evolving speed for each species. We constructed a likelihood ratio test (LRT) using the Codeml program in the PAML package and tested the free ratio model against the fixed ratio model (dN/dS ratios to average). To further identify genes under positive selection, we used a modified branch-site model [68] , in which LRT P -values were computed on the assumption that the null distribution was a 50:50 mixture of a χ 2 -distribution with one degree of freedom and a point mass at zero. Fisher’s exact test was used to test for over-represented KEGG pathways among rapidly evolving and positively selected genes, followed by an FDR multiple testing correction (FDR ≪ 0.05). The background was set to all single-copy genes that passed the ds saturation filter. Pathways containing less than 10 genes were neglected. Immune system analysis In innate immunity, TLRs are molecular sensors that recognize the pathogens, and TNFs, ILs and IFNs are cytokines that mediate immune responses [10] . In adaptive immunity, MHC class I molecules present endogenous antigens to activate CD8 + T cells and MHC class II molecules present exogenous antigens to activate CD4 + helper T cells [10] , [69] . Type II IFN (IFNγ) is initially produced by natural killer cells in innate immunity and then by CD4 + helper T cells and CD8 + T cells in adaptive immunity [43] . We retrieved immunity-related genes in the croaker genome based on our functional annotation results. To confirm the absence of genes encoding CD4, we aligned homologues in other teleost genomes to the croaker genome and transcriptome using tblast (E-value=1 × 10 −5 ) and then joined the high-scoring segment pairs (HSP) using an in-house Perl script and screened for open reading frames (ORF) using GeneWise [70] . Finally, we found a truncated CD4-like gene region in the croaker genome. Multiple protein sequencing alignments were performed using ClustalX with default parameters. qPCR assays were performed to detect the expression level of the CD4-like gene in virus-infected croakers ( Supplementary Note 4 ). β-Actin was used as a control to normalize the expression of each template. The TLR3 gene, which is known to be highly expressed in virus-infected croaker [11] , [12] , was used as a positive control. How to cite this article : Wu, C. et al . The draft genome of the large yellow croaker reveals well-developed innate immunity. Nat. Commun. 5:5227 doi: 10.1038/ncomms6227 (2014). Accession codes: The whole-genome sequencing project for Larimichthys crocea has been deposited in DDBJ/EMBL/GenBank Bioproject database under the accession code JPYK00000000 .